Design rules for self-assembled block copolymer patterns using tiled templates Directed self-assembly of block copolymers has been used for fabricating various nanoscale patterns, ranging from periodic lines to simple bends. However, assemblies of dense bends, junctions and line segments in a single pattern have not been achieved by using sparse templates, because no systematic template design methods for achieving such complex patterns existed. To direct a complex pattern by using a sparse template, the template needs to encode the key information contained in the final pattern, without being a simple copy of the pattern. Here we develop a set of topographic template tiles consisting of square lattices of posts with a restricted range of geometric features. The block copolymer patterns resulting from all tile arrangements are determined. By combining tiles in different ways, it is possible to predict a relatively simple template that will direct the formation of non-trivial block copolymer patterns, providing a new template design method for a complex block copolymer pattern. The self-assembly of block copolymer thin films can generate dense nanoscale patterns over large areas [1] , [2] , [3] , [4] , [5] , [6] , [7] , [8] . When directed by a sparse topographic or chemical template, the block copolymers self-assemble into long-range ordered patterns with a controlled orientation [9] , [10] , [11] , [12] , [13] , [14] , [15] , [16] , [17] . These aligned patterns have been used as lithographic masks to fabricate devices including patterned magnetic recording media, flash memory and nanowire or graphene ribbon transistors [18] , [19] , [20] , [21] , [22] , [23] , [24] , [25] . Aperiodic templates are necessary to fabricate patterns consisting of combinations of bends, line segments and junctions using block-copolymer-directed self-assembly. Stoykovich et al. and Liu et al . [14] , [15] have shown that an array of jogs, bends or T-junctions and an isolated jog can be formed from a self-assembled polystyrene- b -polymethylmethacrylate block copolymer with lamellar morphology on a chemical template. We have shown previously that a polystyrene- b -polydimethylsiloxane (PS- b -PDMS) block copolymer with cylindrical morphology can be directed to form an array of bends by using a topographic template [13] . These approaches rely on the intuitive design of templates that contain features with similar density and arrangement to the features in the target pattern and produce relatively simple and periodic patterns. Recently, we theoretically designed templates for directed self-assembly using a Monte Carlo algorithm to move posts randomly within the simulation cell until the free energy is minimized. By using this method, a template for an array of junctions was predicted [26] , [27] , but the template features were not constrained to have any predetermined spacing or location. What is missing in these three approaches is the ability to template patterns over a large area that contain complex assemblies of dense bends, terminations and junctions directed by a simple (and therefore, more easily manufacturable) template. In this work, we present a general and modular approach to designing and fabricating dense and complex block copolymer patterns by developing block copolymer assembly rules for square template tiles and joining the tiles together in a mosaic to form various complex block copolymer patterns. The template tiles consisted of a restricted set of post motifs. By limiting the number of possible post motifs, we study both experimentally and through simulations the block copolymer patterns and defects generated from all tile combinations as well as interactions between the tiles. Based on these results, we develop a set of template design tiling rules for our system that can be used for designing a template to achieve a complex block copolymer pattern. Development of rules for a square-grid template We first demonstrate that the orientation of block copolymer cylinders can be restricted to two orthogonal in-plane directions by using a square lattice of topographic features. Square lattices of topographic single posts with a pitch of 39 nm were fabricated by means of electron-beam lithography. Next, the substrates and posts were chemically functionalized with hydroxyl-terminated PDMS [28] . A PS- b -PDMS block copolymer with cylindrical morphology was spin-coated onto the substrate, and then solvent-annealed and finally etched to yield oxidized PDMS cylinders. On an unpatterned substrate, the observed equilibrium periodicity of the PDMS cylinders ( L 0 ) was ~39±2 nm. 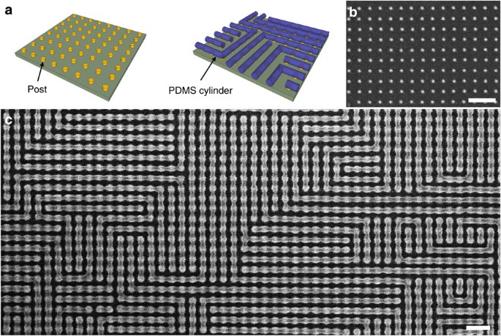Figure 1: PDMS cylinders templated by a square array of posts. (a) Three-dimensional schematic diagram showing how the polydimethylsiloxane (PDMS) cylinders were self-assembled on the post array. (b) SEM image of a square array of posts with a periodicity of 39 nm. The height of the post was 28±1 nm and the diameter was 10±1 nm. (c) SEM image of the PDMS cylinders templated by the post array inb. Since the pitch of the template was commensurate with the block copolymer, two orientations (parallel to thexaxis and to theyaxis) were degenerate and equally probable. Bends or terminations formed where the orientation of the PDMS cylinder changes. Scale bars, 100 nm. Figure 1 shows PDMS cylinders formed on a substrate with a single-post array which had a periodicity that matched L 0 (39 nm). Figure 1b,c shows scanning electron microscopy (SEM) images of the 39-nm periodicity post array and the PDMS cylinders templated by this post array. As shown in Fig. 1c , the block copolymer pattern templated by an array of single posts consisted of many grains (regions of parallel cylinders). The grains were degenerately aligned parallel either to the x axis or to the y axis, since both orientations were equally probable and both directions were commensurate orientations. Bends and terminations formed where two grains with different orientations met. The position of the bends or terminations was random, because the size of the grains was not uniform and also the centre positions of the grains were not evenly spaced. As the templates occupy only a small fraction of the final pattern, fabricating the square lattice of posts instead of the complete pattern of lines would increase the throughput of the lithography process, provided the positions of the bends and terminations can be controlled. Figure 1: PDMS cylinders templated by a square array of posts. ( a ) Three-dimensional schematic diagram showing how the polydimethylsiloxane (PDMS) cylinders were self-assembled on the post array. ( b ) SEM image of a square array of posts with a periodicity of 39 nm. The height of the post was 28±1 nm and the diameter was 10±1 nm. ( c ) SEM image of the PDMS cylinders templated by the post array in b . Since the pitch of the template was commensurate with the block copolymer, two orientations (parallel to the x axis and to the y axis) were degenerate and equally probable. Bends or terminations formed where the orientation of the PDMS cylinder changes. Scale bars, 100 nm. Full size image To control the positions of the bends and terminations, we introduced double posts to the square array of single posts. In previous work, double posts were shown to promote block copolymer cylinders to align parallel to the direction of the double posts [13] . By replacing a single post in the array with a double post, we can locally break the degeneracy of the square array. We replaced one out of every nine single posts with a double post ( Fig. 2a ). We defined the resulting 3-by-3 post array consisting of eight single posts and one double post at the centre as a tile. As a result, a large square array of single and double posts shown in Fig. 2a can be regarded as a checkerboard of tiles. However, the post array can be described equivalently by using another cell, defined as a design cell. As shown in Fig. 2a and the inset of Fig. 2a , a design cell consists of four single posts at the centre and four double posts and eight single posts at the boundary. Because the single and double posts at the boundary are shared with the neighbour design cells, one design cell consists of eight single posts and one double post. Unlike a tile, the block copolymer cylinders formed on the single posts in the design cell (coloured region in the inset of Fig. 2a ) are primarily templated by the four double posts at its boundary. So, the block copolymer pattern of a design cell is primarily determined by the orientations of the surrounding four double posts. The periodicity of the post template defines the periodicity of the final block copolymer pattern, and can be altered slightly (~+/−10%) from L 0 while still effectively templating the block copolymer. 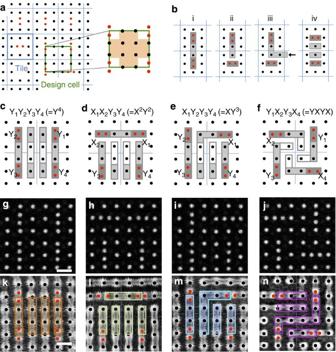Figure 2: PDMS cylinders templated by a square array of posts. (a) Schematic diagram showing templates used in this study. Black dots represent single posts and pairs of red dots represent double posts. The blue box represents a tile and green box represents a design cell. PDMS cylinders formed in a coloured region would be primarily templated by the surrounding four double posts. (b) Schematic diagrams showing how PDMS cylinder patterns on single posts vary depending on the orientations of the closest two double posts. Dark-grey rectangles are the PDMS cylinders assembled on double posts and light-grey rectangles are the PDMS cylinders assembled on single posts. In iii, an arrow represents a PDMS cylinder coming from a neighbouring post. (c–f) Predicted block copolymer patterns of the four different arrangements of a design cell. White rectangles represent predicted block copolymer patterns on four single posts at the centre of a design cell. (g–j) SEM images of the templates of the four arrangements. (k–n) SEM images of the most frequently observed block copolymer patterns formed on the four arrangements. Different colours were used to distinguish the block copolymer patterns from different design cell arrangements. Scale bars, 50 nm. Figure 2: PDMS cylinders templated by a square array of posts. ( a ) Schematic diagram showing templates used in this study. Black dots represent single posts and pairs of red dots represent double posts. The blue box represents a tile and green box represents a design cell. PDMS cylinders formed in a coloured region would be primarily templated by the surrounding four double posts. ( b ) Schematic diagrams showing how PDMS cylinder patterns on single posts vary depending on the orientations of the closest two double posts. Dark-grey rectangles are the PDMS cylinders assembled on double posts and light-grey rectangles are the PDMS cylinders assembled on single posts. In iii, an arrow represents a PDMS cylinder coming from a neighbouring post. ( c – f ) Predicted block copolymer patterns of the four different arrangements of a design cell. White rectangles represent predicted block copolymer patterns on four single posts at the centre of a design cell. ( g – j ) SEM images of the templates of the four arrangements. ( k – n ) SEM images of the most frequently observed block copolymer patterns formed on the four arrangements. Different colours were used to distinguish the block copolymer patterns from different design cell arrangements. Scale bars, 50 nm. Full size image To gain insight into how the PDMS cylinder pattern on a single post in a design cell varies depending on the orientations of the surrounding four double posts, we first studied PDMS cylinders in between two double posts. As shown in Fig. 2b , the PDMS cylinder connected the double posts via the two single posts when the double posts were parallel ( Fig. 2b-i ). The PDMS cylinders made a termination when the two double posts were perpendicular to each other ( Fig. 2b-ii ). However, the PDMS cylinders formed a bend at the single posts instead when another cylinder from a neighbouring post (indicated by an arrow in Fig. 2b-iii ) came into the structure ( Fig. 2b-iii ). When the double posts were aligned parallel to each other in the orthogonal in-plane direction, the PDMS cylinders aligned parallel to the double posts ( Fig. 2b-iv ). By applying the four general observations mentioned above, we predicted the block copolymer pattern templated by each design-cell arrangement. Each double post can be aligned along one of two directions with 16 (2 4 ) possible combinations of the orientations of the four double posts in the design cell. The 16 combinations can be grouped into just four arrangements that are not equivalent under 90° rotations or mirror transformations. Figure 2c–f show the four arrangements and the predicted block copolymer patterns based on the rules described in Fig. 2b . We introduced a notation X 1 X 2 Y 3 Y 4 , in which the first, second, third and fourth letters represent the orientation of the double post in the upper right, upper left, lower left and lower right quadrant, respectively. For a Y 1 Y 2 Y 3 Y 4 (=Y 4 ) arrangement ( Fig. 2c ), the light-grey rectangles connecting dark-grey rectangles on the Y 1 and Y 4 double posts, and the Y 2 and Y 3 double posts were predicted based on the observation in Fig. 2b-i . Light-grey rectangles on the single posts between the Y 1 and Y 2 double posts, and the Y 3 and Y 4 double posts were predicted based on Fig. 2b-iv . After that, white rectangles on the four single posts at the centre of the design cell were predicted to align parallel to the surrounding block copolymer patterns (dark- and light-grey rectangles). For the other three arrangements, the block copolymer patterns were predicted based on the observations in Fig. 2b-i,ii,iv for an X 1 X 2 Y 3 Y 4 (=X 2 Y 2 ) arrangement ( Fig. 2d ), Fig. 2b-i,ii,iii,iv for a X 1 Y 2 Y 3 Y 4 (=XY 3 ) arrangement ( Fig. 2e ) and Fig. 2b-iii for an Y 1 X 2 Y 3 X 4 (=YXYX) arrangement ( Fig. 2f ). In these three arrangements, the patterns on the four single posts at the centre of each design cell were predicted to align parallel to the surrounding block copolymer patterns. When a block copolymer film was annealed with these four design-cell arrangements, the PDMS cylinders formed various patterns on each arrangement. Figure 2k–n show SEM images of the most frequently observed patterns formed on the four arrangements. For Y 1 Y 2 Y 3 Y 4 (=Y 4 ), X 1 X 2 Y 3 Y 4 (=X 2 Y 2 ) and X 1 Y 2 Y 3 Y 4 (=XY 3 ) arrangements, the most frequently observed patterns were identical to the predicted patterns shown in Fig. 2c–e . However, for an Y 1 X 2 Y 3 X 4 (=YXYX) arrangement, the predicted pattern in Fig. 2f was not observed. Instead, several patterns were observed from the YXYX arrangement ( Supplementary Fig. 1 and Supplementary Discussion ), with the one shown in Fig. 2n occurring most frequently. In several experimental trials, the pattern of Fig. 2n was observed in 20% of the YXYX cells. Prediction of patterns formed on a given template To show that the patterns in Fig. 2k–n can be used for predicting the block copolymer pattern formed on a large-area template, we fabricated a square array template of single and double posts and checked whether the final PDMS pattern agreed with the predictions. 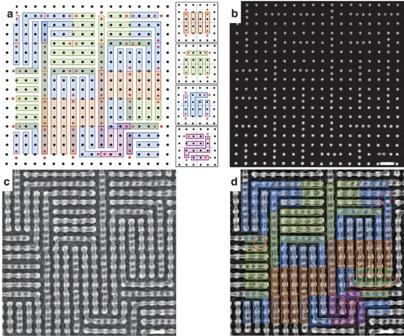Figure 3: Prediction of the PDMS patterns directed by a random template. (a) Random template and the predicted patterns. Insets show the block copolymer patterns of the four design-cell arrangements used for the prediction. (b) SEM image of the fabricated template. (c) SEM image of the PDMS cylinders formed on the template shown inb. (d) The predicted pattern overlaid on the SEM image of the PDMS cylinders. Red circles and ellipsoid indicate mismatches between the prediction and experimental result. Scale bars, 50 nm. Figure 3a shows the test template layout in which the orientations of the double posts in the layout were random. The design cells having Y 4 , X 2 Y 2 , XY 3 and YXYX arrangements were predicted based on the patterns in Fig. 2k–n , as shown in Fig. 3a . When the predicted patterns from two neighbouring design cells conflicted, the pattern was determined by the basic observations shown in Fig. 2b ( Supplementary Fig. 2 and Supplementary Discussion ). Figure 3b shows a SEM image of the template and Fig. 3c shows the PDMS patterns directed by the template of Fig. 3b . To quantify the accuracy of the prediction, we introduced the design-cell prediction yield as D Y% . D Y% was defined as the ratio of the number of completely matched design cells to the total number of design cells. To quantify the degree of similarity between the predicted pattern and observed pattern, we introduced the grid prediction yield G Y% . G Y% was defined as the ratio of the number of matched features on individual grid points to the total number of grid points ( Supplementary Fig. 3 and Supplementary Discussion ). When the predicted pattern was compared with the block copolymer pattern, G Y% =97% (467/480) (more typically G Y% ≈90%) and D Y% =76% (19/25), as shown in Fig. 3d . Red circles and ellipsoid indicate mismatches between the prediction and experimental result. Figure 3: Prediction of the PDMS patterns directed by a random template. ( a ) Random template and the predicted patterns. Insets show the block copolymer patterns of the four design-cell arrangements used for the prediction. ( b ) SEM image of the fabricated template. ( c ) SEM image of the PDMS cylinders formed on the template shown in b . ( d ) The predicted pattern overlaid on the SEM image of the PDMS cylinders. Red circles and ellipsoid indicate mismatches between the prediction and experimental result. Scale bars, 50 nm. Full size image Template design to achieve a target pattern To demonstrate that complex target patterns can be templated by applying appropriate design rules, we fabricated two complex patterns consisting of many bends and terminations. 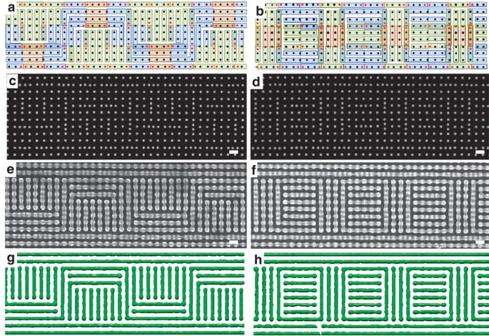Figure 4: Two examples of complex block copolymer pattern fabrication. (a,b) Two template layouts to fabricate complex patterns consisting of dense bends and terminations. Each colour represents the pattern templated by each arrangement. (c,d) SEM images of the templates to fabricate dense patterns of bends and terminations. (e,f) SEM images of the PDMS patterns formed on the template shown incandd.GY%=97% (Fig. 3e) and 99% (Fig. 3f). (g,h) SCFT simulation result showing the constant 50% density surface of PDMS cylinders assembled with the template incandd. Scale bars, 50 nm. Figure 4a,b show the template layouts and the block copolymer patterns predicted to form on these templates. Fig. 4c,d show SEM images of the templates and Fig. 4e,f show the PDMS patterns directed by the templates. Here G Y% =97% ( Fig. 4e ) and 99% ( Fig. 4f ). Furthermore, as shown in Fig. 4g,h , self-consistent field theory (SCFT) simulations [29] , [30] , [31] , [32] , [33] were used to calculate the block copolymer morphology resulting from the input templates of Fig. 4a,b . There is a very good agreement between the structure predicted from the empirically derived design rules, the structure predicted by SCFT and the structure observed in the experiments. The tile-based approach produces a limited range of microdomain arrangements from the four basic template arrangements, and therefore the large area patterns that can be produced by concatenating them are also limited. We expect that a different set of tiles with a greater number of basic geometries would give access to more diverse patterns. The utility of the tile-based approach comes from a compromise between having a template that can produce enough patterns to concatenate into useful structures, while avoiding a template that produces so many patterns that the selectivity between them is too small for design rules to be applicable. Figure 4: Two examples of complex block copolymer pattern fabrication. ( a , b ) Two template layouts to fabricate complex patterns consisting of dense bends and terminations. Each colour represents the pattern templated by each arrangement. ( c , d ) SEM images of the templates to fabricate dense patterns of bends and terminations. ( e , f ) SEM images of the PDMS patterns formed on the template shown in c and d . G Y% =97% ( Fig. 3e ) and 99% ( Fig. 3f ). ( g , h ) SCFT simulation result showing the constant 50% density surface of PDMS cylinders assembled with the template in c and d . Scale bars, 50 nm. Full size image Free energy of various patterns formed on two arrangements To understand the differences between the experiment and prediction shown in Figs 3 and 4 , we fabricated a large template array consisting of various different combinations of tile arrangements and observed the self-assembled patterns of the block copolymer on the template. D Y% was 100% for the Y 4 arrangement having four parallel PDMS cylinders regardless of the arrangement of their nearest neighbour design cells. D Y% =64% for the X 2 Y 2 arrangement having a pattern identical to the predicted pattern, as shown in Fig. 5a-i . However, 7% of the X 2 Y 2 arrangements yielded an internal bend, as shown in Fig. 5a-iii,iv . As shown in Fig. 5a-ii,iii,iv,v , G Y% of the unmatched patterns were 92%, 88%, 79% and 83%, respectively. For the XY 3 arrangement, D Y% was 60%, as shown in Fig. 5b-i . In 13% of the XY 3 arrangements, the position of a bend was shifted by one grid point to the X 1 double post, as shown in Fig. 5b-ii . In 10% of the XY 3 arrangements, the position of a bend was shifted by one grid point to the Y 3 double post, as shown in Fig. 5b-iii . The pattern mismatch in Fig. 5a-ii,iii,iv,v and b-ii,iii,iv resulted from a common defective feature. We expect that the formation of this defect could be reduced by modifying the cell geometry, for example, by using an elliptical post ( Supplementary Fig. 4 and Supplementary Discussion ). 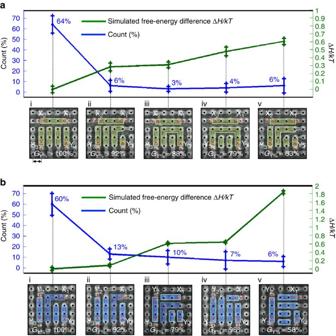Figure 5: Counts and simulated free energy differences of two arrangements. (a,b) Panel i shows the SEM image of the PDMS pattern identical to the predicted pattern ofa, X2Y2arrangement andb, XY3arrangement. Panels ii–v show other patterns observed from thea, X2Y2arrangement andb, XY3arrangement. Error bars show ±1 standard deviation of the count (blue line) and simulated free energy difference (green line).GY%is the grid point yield of each pattern. The ranges of the rightyaxis inaandbare different. Length of double arrow is 39 nm. Figure 5: Counts and simulated free energy differences of two arrangements. ( a,b ) Panel i shows the SEM image of the PDMS pattern identical to the predicted pattern of a , X 2 Y 2 arrangement and b , XY 3 arrangement. Panels ii–v show other patterns observed from the a , X 2 Y 2 arrangement and b , XY 3 arrangement. Error bars show ±1 standard deviation of the count (blue line) and simulated free energy difference (green line). G Y% is the grid point yield of each pattern. The ranges of the right y axis in a and b are different. Length of double arrow is 39 nm. Full size image To gain insight about the relative counts of the patterns shown in Fig. 5 , we used SCFT simulations to compute the free energy of those patterns and investigate the equilibrium stability of the patterns. These free energy comparisons for the five structures seeded for the X 2 Y 2 and XY 3 arrangements are shown in Fig. 5a,b respectively. The general trend here is that the structures observed with a lower frequency had a higher free energy than the structure found most often. The qualitative agreement is good even though the model does not account for several features of the physical system: in particular, the SCFT model does not consider the solvent anneal explicitly but rather implicitly through an effective χ , and does not consider kinetic limitations to the formation of structures. It is also limited to periodic boundary conditions, does not consider fluctuations in film thickness, and the parameters for surface affinity, post geometry and so on are not exact. Although kinetic effects are expected to be relevant, the fact that the less frequently observed structures have higher free energies in the simulation implies that the morphology is primarily driven by thermodynamic considerations. The restricted set of geometric features presented in this study allows one to design a template for fabricating a complex pattern without relying on intuition [13] . The templating effect of one double post is mainly decided by the orientations of its neighbouring double posts, and is therefore restricted to its local surroundings. Predicting a block copolymer pattern from a given template layout or designing a template layout for a target pattern is therefore simplified to just assembling design cells, and we expect that in principle, non-trivial patterns over a large area (for example, a pattern relevant to an integrated circuit layout) could be achieved. This approach to complex templating provides advantages in the context of nanolithography. First, the time required for writing the template using electron-beam lithography can be a factor of five or more shorter than the time required to write the complete pattern ( Supplementary Fig. 5 and Supplementary Discussion ). The throughput could be further increased by using a two-step process for template generation, instead of writing all the posts serially: (1) the basic square array of posts could be fabricated by interference lithography or another massively parallel technique, which can generate periodic patterns over a large area with high throughput and (2) the aperiodic double posts could then be fabricated by electron-beam lithography or by another serial method ( Supplementary Fig. 5 and Supplementary Discussion ). Second, we believe that the four block copolymer patterns shown in Fig. 2k–n are only a subset of block copolymer patterns that could be achieved. We expect that a variety of block copolymer patterns could be achieved by fine-tuning parameters including the height and diameter of the posts and the block copolymer film thickness, volume fraction and annealing conditions. Additional template arrangements could be developed by removing a post or using a triple post or quadruple post instead of a double post. For example, a T-junction was formed reproducibly when a post was missing ( Supplementary Fig. 6 and Supplementary Discussion ). Tiles incorporating such features would extend the rules and the available block copolymer geometries beyond what has been demonstrated here. Third, this approach could be used to achieve a block copolymer pattern with higher resolution. For example, a block copolymer pattern with a periodicity of 18 nm could be achieved by templating a 16 kg mol −1 PS- b -PDMS block copolymer [16] using a square post array with a periodicity of 18 nm and double posts with a post spacing of 12 nm. This resolution is difficult to achieve with electron-beam lithography, but similar resolution has been achieved by helium-ion beam lithography [34] and scanning transmission electron microscopy lithography [35] . In summary, a template design based on a restricted set of tiles with post motifs provides a way to achieve a complex pattern of line segments with bends and terminations from a relatively simple template. Forming a complex block copolymer pattern by concatenating design cells (tiles) derived from a limited number of local template arrangements greatly reduces the difficulty of the template design process and the amount of experimentation required to achieve the target pattern. This approach, starting from a degenerate template, adding a restricted set of perturbations and developing rules for all possible perturbation arrangements, could potentially be applied to other self-assembling systems that can be templated by topographic or chemical features. Rule-based patterning strategies have been developed for other self-assembling systems such as DNA origami [36] , [37] , [38] . In DNA origami, the information used to control the patterning is input via DNA synthesis, and is thus too slow to address the enormous challenge of pattern generation in a modern technological setting (a single mask for the semiconductor industry can take 5 days to pattern at a data input rate of 10 8 bits per second). The application of such rule-based strategies to simple chemical systems, such as block copolymers, potentially solves the modern pattern generation problem, as the information defining the pattern is input lithographically. We expect that rule-based strategies could be developed further to describe assembly of other nanoscale objects such as nanoparticles, for example, by functionalizing or programming nanoparticles with ligands that promote specific types of interactions [39] , [40] . Extensions of the algorithmic strategies described here for block copolymers may enable further levels of control over the final pattern, and ultimately lead to a robust inverse-design process that determines the optimum template for a given target pattern. Template fabrication The templates were fabricated by using electron-beam patterning of hydrogen silsesquioxane (HSQ). HSQ films (XR-1541 2% solids from Dow Corning) with a thickness of 28±1 nm were spin-coated on a silicon substrate. Single-pixel dots were exposed in an Elionix ELS-F125 electron-beam lithography tool at 125 kV acceleration voltage. Square arrays of single dots with a diameter of 10±1 nm and a range of pitches from 30 to 42 nm were exposed. The exposed samples were developed with a salty development system as described previously [41] . The developed sample was treated with O 2 /He plasma (50 W, 10 s) to convert HSQ posts into silicon oxide. To measure the diameter of the templates, SEM images of the templates were obtained by using a Raith 150 scanning electron microscope operated with an acceleration voltage of 10 kV. The errors of the template diameter were estimated from visual inspection of the SEM images. Block copolymer self-assembly The patterned substrates were treated with a hydroxyl-terminated PDMS brush layer (0.8 kg mol −1 , Polymer Source Inc., 170 °C for 12 h) to render the HSQ nano-posts attractive to the PDMS block. Two percent of PS- b -PDMS ( M w =45.4 kg mol −1 , f PDMS =33.5%, Polymer Source Inc.) solution in propylene glycol monomethyl ether acetate was spin coated onto templated substrate to a thickness of 35 nm. The films were solvent annealed using either a flow-controlled solvent annealing system or conventional solvent annealing system for 3 h. In the flow-controlled solvent annealing system, nitrogen gas was bubbled through a liquid reservoir of a 5:1 mixture of toluene and heptane at a flow rate of 10 sccm and diluted by nitrogen gas flow of 0.7 sccm so that the annealing chamber was maintained at constant solvent vapour pressure. The vapour pressure was controlled by changing the flow ratio between the solvent stream and the nitrogen stream [42] . In the conventional solvent annealing system, the sample was placed in a chamber containing a reservoir of liquid solvent (5:1 mixture of toluene and heptane). On an unpatterned substrate, the equilibrium periodicity of the PDMS cylinders ( L 0 ) was ~39±2 nm. Reactive ion etching The annealed block copolymer films were treated with a 50 W, 10 mTorr CF 4 plasma for 5 s and then a 90 W, 6 mTorr O 2 plasma for 22 s to remove the top PDMS surface layer and then the PS matrix. This two-step reactive ion etching process left oxygen-plasma-modified PDMS cylinders on the substrate [13] . The PDMS cylinders were imaged with a Raith 150 SEM operated with an acceleration voltage of 10 kV. SCFT simulation The SCFT simulations used here use the same equations and computational methods as presented in the supporting information of previous work by Mickiewicz et al. [31] In the SCFT simulations, the system was modelled by using hard-wall field boundary conditions that represented the topographic posts used in experiment and PDMS attractive potentials that represented the surface–air interface and brush layer. The system was discretized onto an N x -by- N y -by- N z grid with a course graining of nine grid points assigned to a distance of L 0 . Both 2D ( N Z =1) and 3D simulations were performed for comparison (note that only the final 3D results are reported here). The posts were modelled with a hard-wall potential field value surrounded by an attractive field parameter modelling the PDMS brush layer. Two coarse grainings of posts were used as schematically shown in Supplementary Fig. 7 with the first single-point hard-wall potential corresponding to ~8 nm post and brush layer and the second five-point hard-wall potential corresponding to ~16 nm post and brush layer. These 9-by-9 grids were concatenated to form the entire simulation cells used with periodic boundary conditions imposed in the planar directions and confined boundary conditions in the thickness direction for the 3D simulations. The resulting simulation cells were on the order of ~108 by ~108 by 20 grid points (the thickness here chosen to roughly correspond to a swelling thickness observed in experiment of ~2.0 L 0 ). The lateral grid points used varied depending upon the simulations. Since the primary interest in using the simulations was to explore the energetics of various structures, most simulations were seeded with target structures and the chemical potential fields relaxed holding the seeded density fields constant to obtain estimates of the free energy of the structures. These target structure density fields were created by first simulating a single cylinder feature over a single or double post in a 9-by-9-by-20 grid and then concatenating the field results into the appropriate seed structure. The field relaxation required two steps. First the exchange field Ω − was relaxed until the free energy reached an approximately constant value (~10,000–20,000 iterations). Then the pressure fields Ω + were relaxed based on the density solution of the relaxed Ω − until the free energy was again approximately constant. Various likely seed structures were used to test each template. In the experiment, the film thickness during solvent swelling varied from around 1.5 to 2.0 L 0 , so in the simulations a film thickness corresponding to 2.0 L 0 was chosen for simplicity in 3D simulations, though further studies on the effect of film thickness on the structures and viability of the design rules for these thicknesses should be taken into consideration. The post heights used in the experiment were around ~2/3 L 0 but it has been observed that the exact height in relation to the film thickness affects the final morphology, so various post heights were tried in preliminary simulations. Since the experimental system is solvent annealed, the exact equilibrium volume fraction may not be exactly the bulk value due to the solvent preferentially swelling the two blocks differently. Thus different volume fractions were tried during preliminary simulations. The exact χ -value used was reduced by a factor of ~1/2 since the solvent was modelled implicitly by varying χ and the volume fraction (assuming ~50% of the system consists of solvent). Since all these parameters need to be optimized for comparison with experiment, an initial screening of the structure made experimentally in Fig. 3g was initiated in the simulations for a range of post heights from 0.67 L 0 to 1.11 L 0 and a range of volume fractions from 0.30 to 0.37 on a 162-by-81-by-16 grid. Here the thickness corresponded to 1.5 L 0 . The resulting minority densities after 10,000 iterations were calculated and are shown for the interface density of 0.5 in 3D along with the total energy of the system (not normalized by grid point volume) in Supplementary Fig. 8 . From these simulations, the seeded structure only stabilized for volume fractions >0.35 in the simulation. For all the post heights used, these higher volume fractions kept the structure after relaxing the fields, but the lowest energy structure occurred for the shorter posts. Based on these considerations, the lowest volume fraction that kept the structures intact of 0.36 and height that gave the lowest free energy of 0.78 L 0 were chosen to use as the parameters for free energy comparison simulations of structures observed in the X 2 Y 2 and XY 3 design cells. These parameters do not correspond exactly to the experiment, so other parameters such as total design-cell thickness and surface energy attraction strength could be optimized to get better corresponding results. However, this optimization is not necessary since only general free energy trends were of interest. The surface energy attraction strength was based upon the values used in previous studies [4] . Using the parameters corresponding to stable formation of the target cylindrical patterns, the 10 structures shown in Fig. 4 were each seeded into a simulation box with appropriate X 2 Y 2 and XY 3 template boundary conditions. To eliminate effects of periodic boundary conditions, internal reflective boundary conditions were implemented such that a four-fold reflective simulation cell was created for the structures with additional buffer layers of X 4 or Y 4 design cells that were the same in each simulation for the given boundary conditions. In these simulations, the block copolymer was modelled with a Flory–Huggins parameter χ =0.224, N =125 effective Kuhn monomer segments and volume fraction of f =0.36, and topographic post features modelled as hard wall potential fields surrounded with a preferential surface field to model brush layer surface energies and air-interface surface energies in periodically bound design cells of size 81-by-81-by-20. The density fields that were seeded are shown as 3D isosurface for the 50% interface density between the two blocks in Supplementary Fig. 9 . The difference in the free energy of the structures calculated holding the density fields constant while relaxing the fields and their standard deviation are thus shown in the main text in Fig. 4 . Note that the use of reflective boundary conditions rather than considering neighbouring design cells as well as having a buffer layer of the Y 4 structure may change some of the energetics at the boundary of the structures. Since the connectivity of the cylinders differs only in the design cell of interest across a given post template, one can safely compare the relative free energies of these structures. The absolute values of these energies are not as important since they depend on the boundary conditions used. Ideally one would want to calculate a free energy of an isolated design cell, but because there are always boundary issues at the connections, there are inherently effects due to the neighbouring design cells or whatever boundary conditions are chosen that affects the final energetics of the system. How to cite this article: Chang, J.-B. et al. Design rules for self-assembled block copolymer patterns using tiled templates. Nat. Commun. 5:3305 doi: 10.1038/ncomms4305 (2014).